Dual-polarity plasmonic metalens for visible light Surface topography and refractive index profile dictate the deterministic functionality of a lens. The polarity of most lenses reported so far, that is, either positive (convex) or negative (concave), depends on the curvatures of the interfaces. Here we experimentally demonstrate a counter-intuitive dual-polarity flat lens based on helicity-dependent phase discontinuities for circularly polarized light. Specifically, by controlling the helicity of the input light, the positive and negative polarity are interchangeable in one identical flat lens. Helicity-controllable real and virtual focal planes, as well as magnified and demagnified imaging, are observed on the same plasmonic lens at visible and near-infrared wavelengths. The plasmonic metalens with dual polarity may empower advanced research and applications in helicity-dependent focusing and imaging devices, angular-momentum-based quantum information processing and integrated nano-optoelectronics. The optical lens, as an indispensable tool, has been widely exploited in various scientific communities, and its operation is well understood on the basis of classical optics. Traditionally, reshaping the wavefront of the light relies on gradual phase changes, which are accomplished by either controlling the surface topography or varying the spatial profile of the refractive index. Although diffractive and gradient index lenses bring distinguished functionality in imaging and spectroscopy beyond what can be achieved with refractive optics, their applications are limited by the contrast of the refractive index attainable from conventional materials and methods of fabrication. Metamaterials can usually be engineered to exhibit electromagnetic properties that cannot be found in nature or its constituent components [1] , [2] , [3] , [4] , [5] , [6] , [7] , [8] , [9] , [10] , [11] . Broad applications of metamaterials that have been reported to date include invisibility cloaks [1] , [2] , [3] , [4] , [5] , [6] , negative refraction [7] , [8] , [9] , [10] , subdiffraction imaging [11] and nano-optical circuitry [12] , [13] , [14] . Metamaterials offer a wide range of material properties, thus providing an unconventional alternative to lens design. Based on variable refractive index structures, Luneburg lenses have been demonstrated at microwave [15] , [16] and optical frequencies [17] . Nevertheless, they are far from being feasible in practical applications because manufacturing large index gradients in a controlled manner poses great challenges on nanofabrication. Plasmonic lenses based on nano-aperture or nanoslit arrays with varying geometries in a metal film have been proposed and experimentally demonstrated [18] , [19] , [20] , [21] . For the design of most optical components, including lenses, it is important that the phase change can vary smoothly in the range of [0, 2 π ]. However, in those previously reported works, the phase was acquired accumulatively for waves propagating through plasmonic or photonic waveguide modes supported by the nano-apertures, and the attainable phase range is well below 2 π with realistic thickness of the metal film. Furthermore, it is still a technical challenge to create narrow subwavelength slits with extremely high aspect ratios. Recently, the concept of interfacial phase discontinuities has been proposed [22] and the devices based on this new concept have been demonstrated experimentally at infrared wavelength [22] , [23] . The interface consisted of an array of plasmonic antennas that partially converted the linearly polarized incident light into its cross polarization with a discontinuity in phase for both transmission and reflection. Importantly, the phase variation across 2 π can be readily achieved without sacrificing the uniformity of amplitude. Arbitrary phase profiles along the interface can be realized by varying the geometry of each individual plasmonic antenna. Based on this principle, a linear gradient of the phase discontinuity at the interface was realized, leading to anomalous reflection and refraction described by a generalized Snell’s law [22] , [23] . It was further shown that the phase discontinuities generated by a suitably designed plasmonic antenna interface could be utilized to create a vortex beam upon normal illumination by linearly polarized light [22] . Here, we apply the concept of interfacial phase discontinuity to the design of a novel type of ultrathin flat lens with helicity-dependent polarities. Instead of converting one linear polarization to the other as in previous works [22] , [23] , we consider the abrupt phase change that occurs for circularly polarized (CP) light converted to its opposite helicity. The metamorphosing phase shift, ranging from 0 to 2 π , is realized by a metasurface consisting of an array of plasmonic dipoles with subwavelength separations. By adjusting the orientation angle φ of the individual dipole antennas, we can obtain the required phase shift for the plasmonic lens, as the local abrupt phase change is simply given as Φ=±2 φ , with the sign determined by the combination of the incidence/transmission polarizations, with the + sign for left circular polarization (LCP)/right circular polarization (RCP) and the − sign for RCP/LCP (Methods). Interestingly, the sign of the phase discontinuity can be reversed by controlling the helicity of the input and detected CP light. This suggests that the polarity of a lens that is based on the circular polarization phase discontinuity can be metamorphosed by the helicity of the CP light. Moreover, the purely planar geometry of such lens enables promising integration into other nanodevices by using conventional micro- and nanofabrication processes. Note that a lens with dual polarity operating at far infrared wavelengths was demonstrated previously [24] ; however, polarization-dependent imaging has not yet been observed. Here we demonstrate, for the first time, dual-polarity lens operating at visible wavelength. Specifically, we show the unique dual-polarity nature of the lens by not only observing real and virtual focal points, but more importantly, magnified and demagnified imaging on the same plasmonic metalens. Design and fabrication of the lens In order to focus an incident CP plane wave, the flat lensing surface must undergo a spatially varying phase shift. To achieve the phase profile equivalent to a conventional cylindrical lens, the following expression governs the relationship between the rotation angle φ and the location of dipole antenna x : where k 0 =2 π / λ is the free-space wavevector and f is the focal length of the lens. Note that the + and − sign in equation (1) corresponds to a positive (convex) and negative (concave) polarity, respectively, for a RCP incident wave, and the opposite holds for a LCP incident wave. To implement the proposed dual-polarity lens, the rotation angle of the dipole antennas should vary according to equation (1). 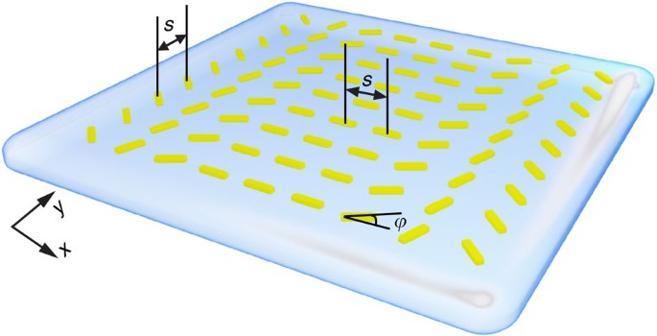Figure 1: Diagram of the bipolar plasmonic lens. The lens consists of an array of plasmonic dipole antennas on a glass substrate with orientations varied along the focusing direction (x). The distance between neighbouring dipoles,S=400 nm, is the same along the two in-plane directions.φis the rotation angle of the dipole relative to thexaxis. The abrupt phase shift is solely determined by the orientation of the dipoles. Figure 1 shows a schematic of the designed plasmonic bipolar lens that consists of dipole nanoantennas with the directional orientation corresponding to a + sign in equation (1). The dipoles are arranged in a two-dimensional array with a subwavelength period of S in both x and y directions. The full-wave numerical validation is performed using a commercial software package (CST Microwave Studio) to simulate the propagation of a CP wave through the plasmonic lens at normal incidence ( Fig. 2 ). In the simulation, we calculated a miniaturized lens, as the size of the fabricated one is beyond the capability of our numerical simulation. The simulated lens in Fig. 2 has a focal length of 10 μm and an aperture of 8 × 8 μm 2 , consisting of 21 dipole antennas along the x direction with S =400 nm. For an incident beam with RCP, the plasmonic lens functions as a converging (positive) lens. Two focal planes are clearly visible at z =±10 μm away from the plasmonic lens surface, as shown in Fig. 2a . There are two real focal points, one for the transmitted beam and the other for the reflected beam, on each side of the plasmonic lens. Thus by manipulation of the phase discontinuity along an interface with a suitably designed dipole antenna array for the incident CP light, a light wave can be fully concentrated. Figure 1: Diagram of the bipolar plasmonic lens. The lens consists of an array of plasmonic dipole antennas on a glass substrate with orientations varied along the focusing direction ( x ). The distance between neighbouring dipoles, S =400 nm, is the same along the two in-plane directions. φ is the rotation angle of the dipole relative to the x axis. The abrupt phase shift is solely determined by the orientation of the dipoles. 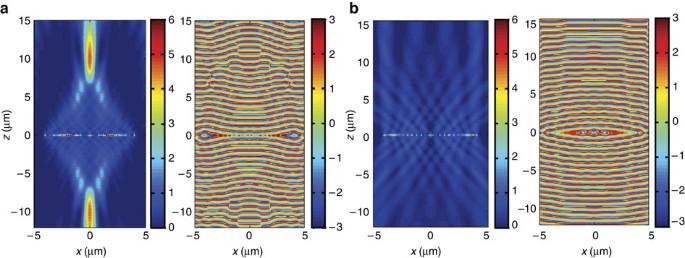Figure 2: Simulation of a dual-polarity plasmonic lens. Full-wave simulations are performed by CST Microwave Studio for the propagation of a CP wave at 740 nm through the lens at normal incidence. (a) Intensity and phase distribution indicate that the lens functions as a positive lens for RCP incident light. (b) With LCP incident light, the same lens changes its polarity and turns into a negative lens. In both plots, only the fields with the circular polarization opposite to that of the incident wave are plotted. Full size image Figure 2: Simulation of a dual-polarity plasmonic lens. Full-wave simulations are performed by CST Microwave Studio for the propagation of a CP wave at 740 nm through the lens at normal incidence. ( a ) Intensity and phase distribution indicate that the lens functions as a positive lens for RCP incident light. ( b ) With LCP incident light, the same lens changes its polarity and turns into a negative lens. In both plots, only the fields with the circular polarization opposite to that of the incident wave are plotted. Full size image When the polarization of the input light is switched from RCP to LCP, the simulation shows that the polarity of the proposed dual-polarity lens is indeed transformed from positive (convex) to negative (concave). This is clearly indicated by the spatial distribution of the intensity and the phase ( Fig. 2b ). Unlike conventional cylindrical lenses, a single flat lens can be metamorphosed to converging and diverging lenses, which only depends on the helicity of the CP light. Based on the interfacial phase discontinuity, we designed and fabricated two plasmonic metalenses, Lens A and Lens B, with a negative and a positive polarity for an incident beam with RCP polarization, respectively. The plasmonic dipole antennas are fabricated by electron-beam lithography on an indium-tin-oxide (ITO)-coated glass substrate. The dipole antennas are made from gold with a thickness of 40 nm. Scanning electron microscopy images for the resulting patterns for Lens A and Lens B designed at 740 nm are shown in Fig. 3a . Each lens has an aperture of 80 × 80 μm 2 and a focal length f A =−60 μm and f B =+60 μm for an incident wave with RCP polarization, respectively. The dipole antennas are 200 nm long and 50 nm wide, exhibiting a longitudinal resonance around 970 nm and a transverse resonance around 730 nm. The rotation angles for the dipoles far from the lens centre change more rapidly than those near the centre. 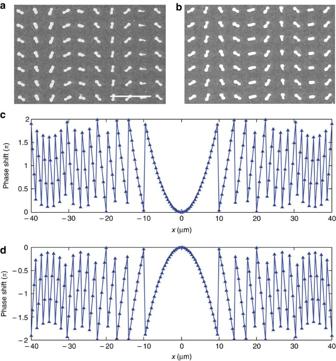Figure 3: Scanning electron microscopy images of selected areas of the plasmonic lenses and the expected profile of phase discontinuity. Scanning electron microscopy images of a plasmonic lens on an ITO-coated glass substrate with (a) negative polarity (Lens A) and (b) positive polarity (Lens B) for an incident light with RCP. The scale bar represents 1 μm. (c,d) The expected phase discontinuity for the positive and negative lens, respectively, for RCP incidence. Note that for LCP incidence, the phase discontinuity is reversed. Figure 3c give the expected abrupt phase changes for the two lenses for RCP incidence, which show opposite phase profiles owing to the opposite rotation directions of the dipole antennas in these two lenses. Figure 3: Scanning electron microscopy images of selected areas of the plasmonic lenses and the expected profile of phase discontinuity. Scanning electron microscopy images of a plasmonic lens on an ITO-coated glass substrate with ( a ) negative polarity (Lens A) and ( b ) positive polarity (Lens B) for an incident light with RCP. The scale bar represents 1 μm. ( c , d ) The expected phase discontinuity for the positive and negative lens, respectively, for RCP incidence. Note that for LCP incidence, the phase discontinuity is reversed. Full size image Characterization of the lens We experimentally demonstrate the performance of the focusing of the plasmonic lens by using a CP laser beam at the wavelength of 740 nm (measurement setup shown in Methods). A positive lens causes the incident laser beam to converge at a focal plane on the transmission side of the lens forming a real focus line, while a negative lens causes the incident laser beam to emerge from the lens as though it is emanated from a virtual focal plane on the incident side of the lens. In the measurement, by gradually adjusting the distance between the objective and the plasmonic lens, we are able to examine the optical intensity distribution at different z locations along the propagation direction to determine the focal plane. 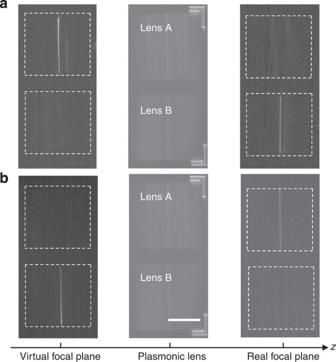Figure 4: Lens polarity is reversed by changing the handedness of the incident light. Optical microscope images at virtual focal plane (left), lens surface (middle) and real focal plane (right) for the incident light with (a) RCP and (b) LCP. CP laser beam is incident on the plasmonic lens from the left along thezdirection, and the lens is located atz=0. Positions of lenses are marked by the white dashed squares The scale bar is 50 μm. The polarity of Lens A is different from that of B for the same CP light. The distance between the real focal plane and the lens is measured to be 60 μm, which is the real focal length. The distance between the real focal plane and the virtual one is 121 μm, which corresponds to 2f. The wavelength of the incident laser beam used in the above images is 740 nm. Figure 4 shows the optical microscopy images for two different incident/transmission polarization combinations: RCP/LCP ( Fig. 4a ) and LCP/RCP ( Fig. 4b ). As shown by Fig. 4a (left) for the RCP incident beam, we observe a bright focused line along the y direction for Lens A at z =−61 μm, which agrees well with the designed focal length. This is a virtual focal point as it lies on the incident side of the plasmonic lens. Hence, it verifies that Lens A is a negative (concave) lens for RCP incident light. On the other hand, a bright focused line is observed for Lens B on the transmission side of the plasmonic lens at z =60 μm, which corresponds to the real focal plane. This confirms that Lens B is positive (convex) for the incident light with RCP polarization. When the polarizations of the incident and transmitted beams are switched to LCP and RCP, respectively, the focusing behaviour for both Lens A and Lens B are reversed, as shown in Fig. 4b . At the virtual focal plane z =−61 μm, a virtual focused line is observed for Lens B and at the real focal plane z =60 μm, a real focal line is observed for Lens A. The conversion in the focusing properties from positive (negative) to negative (positive) is solely attributed to the handedness change of the CP for the incident light, which agrees perfectly with the theoretical prediction. Figure 4: Lens polarity is reversed by changing the handedness of the incident light. Optical microscope images at virtual focal plane (left), lens surface (middle) and real focal plane (right) for the incident light with ( a ) RCP and ( b ) LCP. CP laser beam is incident on the plasmonic lens from the left along the z direction, and the lens is located at z =0. Positions of lenses are marked by the white dashed squares The scale bar is 50 μm. The polarity of Lens A is different from that of B for the same CP light. The distance between the real focal plane and the lens is measured to be 60 μm, which is the real focal length. The distance between the real focal plane and the virtual one is 121 μm, which corresponds to 2 f . The wavelength of the incident laser beam used in the above images is 740 nm. Full size image The major functionality of a lens is imaging. The performance of the plasmonic lens is subsequently explored by the imaging of a chromium grating positioned a distance away from the plasmonic lens. The schematic of the imaging system is given in Fig. 5a . The chromium grating has a pitch of 10 μm and a width of 5 μm. The grating and the lens are separated by a 20-μm-thick air gap. A positive lens for RCP (Lens B type) with a focal length of 60 μm designed for 810 nm is fabricated and characterized for imaging. As the object is within the focal distance, only virtual images are expected for the same lens for both circular polarizations. However, the virtual images show opposite magnifications with respect to the different polarizations of the incident beams, as schematically illustrated by Fig. 5b . Hence, we expect to obtain a magnified and reduced virtual image for the positive lens (RCP incidence) and the negative lens (LCP incidence), respectively. Based on the simple geometrical optics calculation for lenses with focal lengths of ±60 μm, the two virtual image planes are calculated to be at z =−30 μm for the positive lens (RCP incidence) and z =−15 μm for the negative lens (LCP incidence), with a magnification of 1.5 and 0.75, respectively. Experimental imaging results for the two circular polarizations are shown in Fig. 5d . Compared with the image of the grating without the plasmonic lens, magnified and shrinked images formed by the plasmonic lens are indeed observed for different circular polarizations. The magnifications of the gratings in the middle and the bottom of Fig. 5d are 1.45 and 0.87, respectively, which show reasonable agreement with the predicted values. 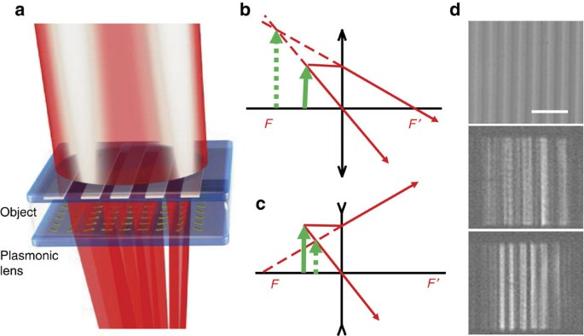Figure 5: Experimental demonstration of polarization-dependent imaging. (a) Schematic of the imaging system. A grating serves as the object. The object and the lens (type B) are separated by an air gap of 20 μm. (b,c) Schematic illustration of imaging for a convex lens (b) and a concave lens (c). (d) Optical microscopy images of the grating at 810 nm without the plasmonic lens (top), a magnified image for RCP incident beam with a magnification of 1.45 (middle) and a reduced image for LCP incident beam with a magnification of 0.87 (bottom). The calculated magnifications based on ray optics are 1.5 and 0.75, respectively. The scale bar is 50 μm. Figure 5: Experimental demonstration of polarization-dependent imaging. ( a ) Schematic of the imaging system. A grating serves as the object. The object and the lens (type B) are separated by an air gap of 20 μm. ( b , c ) Schematic illustration of imaging for a convex lens ( b ) and a concave lens ( c ). ( d ) Optical microscopy images of the grating at 810 nm without the plasmonic lens (top), a magnified image for RCP incident beam with a magnification of 1.45 (middle) and a reduced image for LCP incident beam with a magnification of 0.87 (bottom). The calculated magnifications based on ray optics are 1.5 and 0.75, respectively. The scale bar is 50 μm. Full size image The amount of coupled power between the two circular polarization states is an important aspect in the performance of the lens. For our presented work, the conversion power between the polarization states is measured around 5%. Although this value might be at the lower edge of what is required for practical applications, this relatively low value is due to a technical issue rather than a fundamental limit. With further optimization in the designs, for example, by increasing the density of the dipoles, and better alignment of the resonance wavelength of the antennas to the operating wavelength of the lens, the dipole antennas can achieve a significantly higher transmission in the converted polarization. Here, we have proposed and experimentally realized a plasmonic flat lens with dual polarity operating at visible frequencies. The design is based on the interfacial phase discontinuity that occurs when a CP light is converted into the opposite circular polarization. By controlling the polarizations of the incident and transmitted beams, we show that the focussing properties of the same plasmonic lens can be altered between a convex lens and a concave lens, as in stark contrast to conventional lenses with a fixed polarity. Although a plasmonic lens with dual polarity based on nanoslit array was previously claimed [21] , there was no direct experimental observation of the concave lensing effect, that is, presence of virtual focal plane or demagnified virtual image of an object formed by the plasmonic lens. In contrast, we have unambiguously shown both the convex and concave functionalities of the same plasmonic lens by observing focusing at real and virtual focal planes, and the magnified and demagnified image when an object is placed close to the lens. As the plasmonic lens is made of simple plasmonic dipoles with variable orientation, it does not involve complicated design of plasmonic nanostructures. The dual-polarity plasmonic flat lens opens an avenue for new applications of phase discontinuity devices, and could also have an impact on integrated nanophotonic devices. Upon submission of our work, we noticed the publication of another work on a plasmonic lens based on the same mechanism of abrupt phase discontinuity introduced by a monolayer of plasmonic structures [25] . However, as the phase discontinuity arises from the conversion between linear polarizations, such a plasmonic lens does not exhibit dual polarity. Phase discontinuity in circular polarization basis Consider a light field that is normally incident on a dipole with its orientation direction forming an angle ψ with the x axis. The electric dipole momentum of the single dipole induced by the incident electric field can be expressed as: where p x , p y , E x and E y are the components of the electric dipole momentum and the electric field along x and y direction, and α e is the electric polarizability. For normal incidence, the dipole momentum in equation (2) with an incident CP state can be decomposed into two different CP states with a phase shift of 0 and exp(± i 2 φ ), respectively, where the subscripts R and L indicate the right and left handedness of the CP light, e x and e y represent the unit vectors along the x and the y directions, and represents the unit vector for left-handed (+) and right-handed circular polarization (−), respectively. Thus, for an incident beam with a circular polarization, the radiation from the dipole into the opposite radiation in the forward direction experiences a phase discontinuity Φ=±2 φ , with the sign depending on the combination of the incidence/transmission polarization combinations, + for LCP/RCP and − for RCP/LCP. The abrupt phase change can cover the phase shifts from 0 to 2 π , as φ being tuneable from 0 to π . The sign of the phase shift can be switched between positive and negative when changing the handedness of the incident light. Hence, the polarity of the lens will be changed accordingly. Measurement setup The samples are fabricated on an ITO-coated glass substrate with standard electron-beam lithography, subsequent deposition of 40 nm gold and lift-off processes. 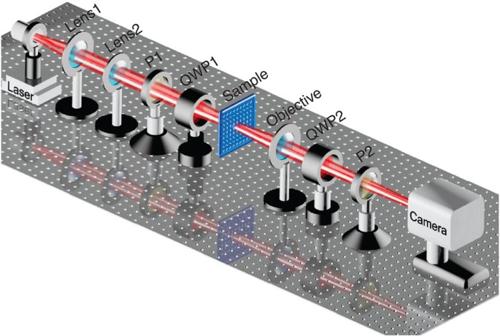Figure 6: Schematic of the optical measurement setup. The polarization directions of the two polarizers are parallel to each other. The incident CP light is generated by the linear polarizer P1 and the QWP1. The opposite circular polarization in transmission is detected by a QWP2 and the linear polariser P2. The microscope objective is mounted on a three-dimensional stage. To image an object, light from a white laser source is incident on the backside of the lens. The transmission through the sample (object and plasmonic lens) is collected with a original magnification X20/0.40 objective and imaged on a charge-coupled device camera. Figure 6 shows the schematic of the optical measurement setup, including several lenses, two quarter-wave plates (QWPs), two linear polarisers, an objective and a charge-coupled device camera. The polarization directions of the two polarisers are parallel to each other. The incident CP light and the opposite circular polarization in transmission are generated by a QWP and a polariser on each side of the plasmonic lens. For the imaging measurement, the microscope objective is mounted on a three-dimensional stage. To image an object, light from a laser source at a wavelength of 740 or 810 nm is incident on the backside of the lens. The transmission through the sample (object and plasmonic lens) is collected with a X20/0.40 objective and imaged on a charge-coupled device camera. Figure 6: Schematic of the optical measurement setup. The polarization directions of the two polarizers are parallel to each other. The incident CP light is generated by the linear polarizer P1 and the QWP1. The opposite circular polarization in transmission is detected by a QWP2 and the linear polariser P2. The microscope objective is mounted on a three-dimensional stage. To image an object, light from a white laser source is incident on the backside of the lens. The transmission through the sample (object and plasmonic lens) is collected with a original magnification X20/0.40 objective and imaged on a charge-coupled device camera. Full size image How to cite this article: Chen, X. et al . Dual-polarity plasmonic metalens for visible light. Nat. Commun. 3:1198 doi: 10.1038/ncomms2207 (2012).